Atomic-scale evolution of modulated phases at the ferroelectric–antiferroelectric morphotropic phase boundary controlled by flexoelectric interaction Physical and structural origins of morphotropic phase boundaries (MPBs) in ferroics remain elusive despite decades of study. The leading competing theories employ either low-symmetry bridging phases or adaptive phases with nanoscale textures to describe different subsets of the macroscopic data, while the decisive atomic-scale information has so far been missing. Here we report direct atomically resolved mapping of polarization and structure order parameter fields in a Sm-doped BiFeO 3 system and their evolution as the system approaches a MPB. We further show that both the experimental phase diagram and the observed phase evolution can be explained by taking into account the flexoelectric interaction, which renders the effective domain wall energy negative, thus stabilizing modulated phases in the vicinity of the MPB. Our study highlights the importance of local order-parameter mapping at the atomic scale and establishes a hitherto unobserved physical origin of spatially modulated phases existing in the vicinity of the MPB. Phase transitions in solids can often be described through order-parameter-based thermodynamic theories, necessitating that the relationship between the order parameter and lattice instabilities is found. For ferroic materials, the nature of the order parameter can be deduced from classical group theory, and relevant structural and dynamical information underpinning the phenomenon can be extracted through elastic and inelastic scattering methods. However, for materials with competing or multidimensional order parameters, the competition between close ground states often results in mesoscopic structural instabilities and associated complex nanoscale morphologies. Examples include monoclinic phases in the vicinity of morphotropic phase boundaries (MPBs) [1] , [2] in ferroics and ferroelectric–antiferroelectric (FE–AFE) boundaries [3] ,correlated oxides [4] and martensites [5] , [6] , [7] . Beyond the fundamental interest, these materials often exhibit striking physical properties, including giant magnetoresistance in phase separated oxides, ultra-large electromechanical coupling coefficients in ferroelectric relaxors [8] , [9] and morphotropic materials, and giant magnetoelectric coupling in birelaxors [10] . The majority of MPB-related studies focus on systems with FE–FE boundaries (for example, Pb(Zr, Ti)O 3 ) owing to their relevance to applications. The two most common theoretical descriptions of MPB phenomena that have emerged from these studies are based on, respectively, the existence of MPB-specific low-symmetry bridging phases [11] , and adaptive phases with nanoscale textures [12] formed by coexisting domains of different phases and ferroic variants due to the vanishingly small domain wall/interface energy close to the MPB. Each one of these theories explains a subset of macroscopic and microscopic observations of these systems, but the ultimate validity test should be that they reproduce the order-parameter field behaviour as observed on the local (atomic) level. Until recently, spatially resolved studies were limited to direct mesoscopic imaging of the nanophase domains [13] , [14] , [15] , [16] , or nanodiffraction experiments in transmission electron microscopes [17] . Such methods provide information on symmetry and misorientation of the nanodomains with respect to each other. However, the detailed internal structure of the network of domains, and in particular, the size and the precise atomic arrangement of boundaries between them cannot be addressed with diffraction-based or mesoscopic approaches. As a result, the structure of the order-parameter fields, their coupling and the nature of the ground state phase that are central to understanding the atomistic mechanisms behind the unique properties of MPB materials have remained unexplained. Here, we report direct atomically resolved mapping of polarization and structure order-parameter fields at the FE–AFE boundary. As a model system, we have chosen Sm-substituted BiFeO 3 (BFO). While this system has an FE–AFE MPB, it bears many similarities to the FE–FE systems. On one hand, while no polarization rotation is involved at the MPB, a direct R 3 c (FE)– Pnma (AFE) phase transition is symmetry-prohibited, suggesting a possibility of a bridging phase; on the other hand, transmission electron microscopy (TEM) studies reported a large degree of local disorder and coexistence of different phases, thus establishing an adaptive phase scenario as another possibility. The universal phase diagram of rare-earth-substituted BFO has been extensively studied using a combination of ferroelectric characterization, piezoresponse microscopy [18] , scattering [19] and TEM [3] , [20] . This article aims to bridge the gap by combining atomic-scale order-parameter mapping with advanced theoretical analysis. Our results—on the macroscopic and the atomic scale—are consistent with a description suggesting that the presence of the flexoelectric interactions renders the effective domain wall energy negative, thus stabilizing modulated phases in the vicinity of the MPB as the thermodynamic ground state of the system. Atomic configuration across the MPB In the present study, the (Bi,Sm)FeO 3 system serves as a particularly versatile platform. At 12%≤[Sm]<14%, the material displays a nano-mixture of FE/AFE phases as previously revealed by TEM, where the rhombohedral R 3 c bulk matrix coexists with regions with pronounced fourfold ordering of the unit cell indicating the presence of a PbZrO 3 -type antiferroelectric structure. At [Sm]=14%, the system is at a MPB exhibiting a transition between the rhombohedral R 3 c phase FE at lower ([Sm] <14%) concentration to the orthorhombic Pnma phase at higher ([Sm]≥14%) concentrations. The corresponding phase diagram is shown in Fig. 1a (ref. 19 ). As the fourfold ordered phase is only present at the compositions close to the MPB (the composition region in light blue in the Fig. 1a ), it can be concluded that this structural phase is either the bridging phase in the sense discussed above, or at the very least an important component of the nanocomposite that is the bridging phase. Previously, we have shown that the fourfold phase has an antipolar nature [21] . 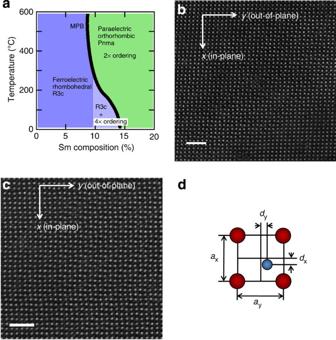Figure 1: STEM studies of the Sm-substituted BFO. (a) Phase diagram showing the ranges of compositional stability of different phases. Reproduced with permission from ref.19(John Wiley and Sons). (b,c) HAADF STEM images of the (b) 10% and (c) 14% Sm-substituted BFO in the ¼[110] ordered AFE region. (d) Schematics of the image quantification technique employed. Bi atoms are represented by red circles, Fe atom is represented by a blue circle. Scale bars are 2 nm. Figure 1: STEM studies of the Sm-substituted BFO. ( a ) Phase diagram showing the ranges of compositional stability of different phases. Reproduced with permission from ref. 19 (John Wiley and Sons). ( b,c ) HAADF STEM images of the ( b ) 10% and ( c ) 14% Sm-substituted BFO in the ¼[110] ordered AFE region. ( d ) Schematics of the image quantification technique employed. Bi atoms are represented by red circles, Fe atom is represented by a blue circle. Scale bars are 2 nm. Full size image Before discussion of the atomic level structural imaging of this material, we briefly note that phase diagrams similar to that in Fig. 1a are universally observed at the morphotropic boundaries between the two ferroelectric phases (for example, monoclinic M phase in lead zirconate titanate) [2] and FE–AFE boundaries. Here, we define the antiferroelectric phase following Tagantsev [22] as a material with competing structural and polarization order parameters, in which structural instability suppresses the polarization. Hence, the FE–AFE transition corresponds to the critical value of structural order parameter at which the state with the total polarization P =0 becomes stable. The application of electric field naturally stabilizes a polarized state, giving rise to classical double hysteresis loops. Thus, the green region in Fig. 1a that shows electric-field induced paraelectric–ferroelectric phase transition accompanied by the double hysteresis loop can be classified as an AFE phase [19] . To gain insight into atomistic mechanisms behind the transition, the microstructure of the substituted BFO was imaged using aberration-corrected scanning transmission electron microscopy (STEM). We focused our attention on the fourfold-modulated phase for antiferroelectric (10% Sm) and MPB (14% Sm) compositions. The films are relaxed and expected to exhibit bulk-like behaviour (see Methods for growth details). Shown in Fig. 1b and c are the high-angle annular dark field (HAADF) image of the 10 and 14% substituted sample in the [100] pseudocubic orientation, respectively. For both ( Fig. 1b and c ), the substrate interface is outside the field of view of the images and oriented vertically. For quantitative structure evaluation, the atomic positions were refined from the raw images (see refs [23] , [24] for details). Local lattice spacing maps were then generated for both Bi/Sm and Fe sublattice (by calculating distances between atoms of the same types), and cation displacement maps were also generated by calculating shifts of the atoms of one type from centres of unit cells formed by atoms of the other type. For BFO, the O sublattice deforms with the Fe sublattice, and thus cation displacement is proportional to polarization [25] , [26] , [27] ; in this article, we refer to polarization behaviour when discussing cation displacements. The analysis procedure is illustrated in Fig. 1d . In the lattice parameter and displacement analysis of the fourfold-modulated phases, no difference in behaviour was found between measurements along the interface (in-plane of the film ( x ), or vertical in Fig. 1 ) and normal to the interface (out-of-plane of the film ( y ), or horizontal in Fig. 1 ), in agreement with the fact that the film is fully relaxed. We will thus limit our discussion to one set of lattice coordinates only, namely, out-of-plane ( y ). Note that in this coordinate system, the electron beam is propagating in z direction. 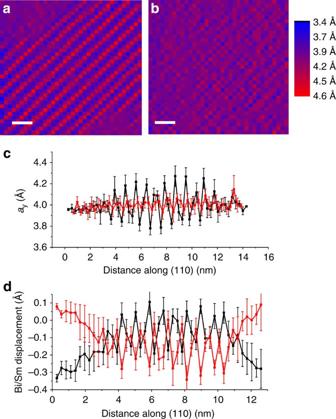Figure 2: Local behaviour of the out-of-plane lattice spacings in 10% Sm-substituted BFO. (a,b) Two-dimensional spacing maps derived from the same HAADF STEM image for (a) Bi/Sm sublattice and (b) Fe sublattice (colour scale applies to both maps). Scale bar is 2 nm. (c) Diagonal profiles of the maps in (a) (black) and (b) (red). Error bars are given as s.d. and reflect variability within an atomic row of the map. Note that Fe spacings have similar variation in ordered and disordered regions, while Bi/Sm spacings are strongly modulated only in the ordered region. In-plane lattice spacings change 180° out of phase with out-of-plane spacings but otherwise show identical behaviour. (d) Diagonal profiles of the relative Bi/Sm displacements calculated from the position data: black—out-of-plane (dy) and red—in-plane (dx). Error bars are given as s.d. and reflect variability within atomic rows of the corresponding maps. Figure 2a and b show two-dimensional maps of out-of-plane lattice spacings calculated from Fig. 1b (10% Sm sample) for Bi/Sm and Fe sublattices. A considerable modulation of the Bi/Sm spacings in the [110] direction is observed in the central area of the map in Fig. 2a (as high as ±6%), while upper left and lower right corners have uniform spacings, showing the coexistence of the modulated AFE phase and parent FE phase. In contrast, the map of Fe spacings in Fig. 2b appears quite featureless, suggesting uniform spacings for both modulated and unmodulated areas. The maps were averaged in a diagonal direction to produce the profiles in Fig. 2c , which show that for Fe spacings, the variations in lattice spacings are indeed uniform across the image (the small ±1% modulation is within the measurement error), while for Bi/Sm spacings, the modulations in the ordered region are very significant. The profile also appears to show regions with intermediate levels of modulation between ordered and disordered phases, but a comparison with the map in Fig. 2b suggests that it is due to the presence of both ordered and disordered regions in these atomic rows. Figure 2: Local behaviour of the out-of-plane lattice spacings in 10% Sm-substituted BFO. ( a,b ) Two-dimensional spacing maps derived from the same HAADF STEM image for ( a ) Bi/Sm sublattice and ( b ) Fe sublattice (colour scale applies to both maps). Scale bar is 2 nm. ( c ) Diagonal profiles of the maps in ( a ) (black) and ( b ) (red). Error bars are given as s.d. and reflect variability within an atomic row of the map. Note that Fe spacings have similar variation in ordered and disordered regions, while Bi/Sm spacings are strongly modulated only in the ordered region. In-plane lattice spacings change 180° out of phase with out-of-plane spacings but otherwise show identical behaviour. ( d ) Diagonal profiles of the relative Bi/Sm displacements calculated from the position data: black—out-of-plane ( d y ) and red—in-plane ( d x ). Error bars are given as s.d. and reflect variability within atomic rows of the corresponding maps. Full size image Given that the Fe sublattice appears undistorted, it is crystallographically more reasonable to talk about Bi/Sm displacements, which we calculated relative to the Fe positions. In Fig. 2d both in-plane and out-of plane displacements are shown, and in the modulated regions, they are out-of-phase, so that the polarization vector is always along the walls of the quadrupled-(110) domains in the ordered area, which are thus uncharged. Given that the Bi/Sm sublattice carries >2/3 of the mass, it is reasonable to define a structural order parameter as the Bi/Sm spacing. Thus, in the fourfold phase for this composition, both structural and polarization order parameters are modulated. Neither the lattice nor polarization is modulated outside of the ordered area, and the displacements tend towards non-zero values, confirming a ferroelectric character of the unmodulated matrix. A similar analysis was performed on a composition directly at the MPB (at Sm 14%), with remarkably different results. The corresponding STEM image is shown in Fig. 1c , while the Bi/Sm and Fe lattice spacing images and corresponding profiles are shown in Fig. 3 . In this image, recorded in a uniformly ordered area, both Bi/Sm and Fe sublattice spacings appear modulated. In fact, the profile in Fig. 3c shows that they are exactly in phase with each other and have comparable moduli. The modulation amplitude for the Bi/Sm sublattice is identical to that observed for the 10% pre-MPB composition ( Fig. 2c ). 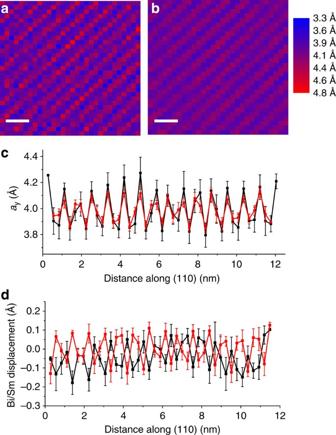Figure 3: Local behaviour of the out-of-plane lattice spacings in 14% Sm-substituted BFO. (a,b) Two-dimensional spacing maps derived from the same HAADF STEM image for (a) Bi/Sm sublattice and (b) Fe sublattice (colour scale applies to both maps). Scale bar is 2 nm. (c) Diagonal profiles of the maps in (a) (black) and (b) (red). Owing to stacking faults in the image, lower left corner was excluded from both profiles. Error bars are given as s.d. and reflect variability within an atomic row of the map. In-plane lattice spacings change 180° out of phase with out-of-plane spacings but otherwise show identical behaviour. (d) Diagonal profiles of Bi/Sm displacements calculated from the position data: black—out-of-plane (dy) and red—in-plane (dx). Error bars are given as s.d. and reflect variability within atomic rows of the corresponding maps. Figure 3: Local behaviour of the out-of-plane lattice spacings in 14% Sm-substituted BFO. ( a,b ) Two-dimensional spacing maps derived from the same HAADF STEM image for ( a ) Bi/Sm sublattice and ( b ) Fe sublattice (colour scale applies to both maps). Scale bar is 2 nm. ( c ) Diagonal profiles of the maps in ( a ) (black) and ( b ) (red). Owing to stacking faults in the image, lower left corner was excluded from both profiles. Error bars are given as s.d. and reflect variability within an atomic row of the map. In-plane lattice spacings change 180° out of phase with out-of-plane spacings but otherwise show identical behaviour. ( d ) Diagonal profiles of Bi/Sm displacements calculated from the position data: black—out-of-plane ( d y ) and red—in-plane ( d x ). Error bars are given as s.d. and reflect variability within atomic rows of the corresponding maps. Full size image Bi/Sm displacement profiles for the MPB composition ( Fig. 3d ) are also quite different from those for the 10% case. While in-plane ( x ) and out-of plane ( y ) displacements remain out-of-phase, thus preserving the polarization orientation along the walls of the quadrupled-(110) domains, the moduli of the displacements are much lower (amplitude decreases by almost 50% compared with that in Fig. 2d ), suggesting that distortions in the Fe sublattice are starting to neutralize polarization (for easy comparison, Figs 2d and 3d are displayed with the same absolute scale). Thus, for this composition, both structural and polarization order parameters are still modulated, but the amplitude for polarization modulation is substantially reduced. EXAFS observations To corroborate the STEM studies and gain insight into the valence states and the site symmetry, we have used soft X-ray near-edge absorption fine structure (NEXAFS) at Sm-M, Fe-L and O-K edges [28] . For the present experiment, we investigated 10% Sm-BFO (pre-MPB), a MPB sample similar to the second STEM sample above, and 15% substituted Sm-BFO (green region in Fig. 1a ), which only shows the orthoferrite structure. While 10% Sm and MPB compositions contain small fractions of other phases, the fourfold-modulated phase is dominant in both, and the results are thus directly comparable to STEM observations. Shown in Fig. 4a and b are the Fe-L and O-K edges spectra obtained under grazing angle conditions. While no significant changes are observed in Sm-M NEXAFS signatures, the Fe-L III of the MPB sample is significantly broader and lower in energy than that of the 10% Sm and 15% Sm samples, consistent with the modulated Fe sublattice in Fig. 3 (see inset on Fig. 4a ). The O-K spectra in the case of the MPB sample also show significant changes, both with respect to bulk undoped BFO [25] , [29] and to compositions with other Sm concentrations. The NEXAFS spectra for the pure BFO have two pre-edge features at ~530 and ~531 eV due to the O 2 p hybridization with unoccupied Fe 3 d minority-spin t 2 g and e g , respectively, a peak at s534 eV due to hybridization between oxygen 2 p and Bi 6 sp states, and a large broad peak with Bi 6 d features at 540 eV [30] , [31] . The 534 eV peak for both the 10% Sm (pre-MPB) and MPB samples are much broader than that of pure BFO, consistent with the distorted Bi sublattice observed in Figs 2 and 3 . For 15% Sm substitution, the Bi 6 sp peak is sharper than that for pre-MPB and MPB compositions (although still broader than that of the pure BFO) as manifested by the deeper valley at 532.5 eV. An extra feature develops at 536 eV associated with the orthorhombic Pnma structure due to the larger ionic radius, as predicted by calculations [29] . The modulation of Fe spacings at the MPB apparently undermines the symmetry of local FeO 6 octahedron, and consequently leads to a weaker Fe3 d -O2 p hybridization. This weaker hybridization is manifested by the red shift of Fe-L-edge at MPB ( Fig. 4a ) and the simultaneous blue shift of the O K-pre-edge (the inset of Fig. 4b ). We note here that a more in-depth analysis of spectral features should be possible once the full structure of the modulated phase, including the details of the octahedral tilt behaviour, is known, enabling theoretical modelling. 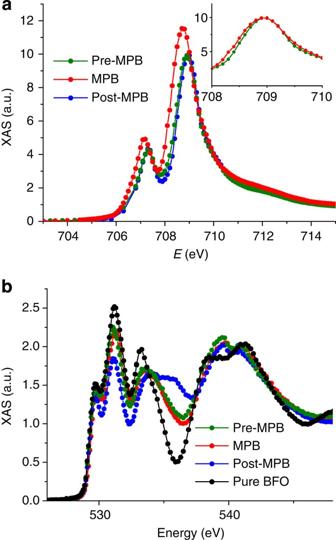Figure 4: NEXAFS data on Sm-substituted BFO samples with different compositions. Pre-MPB (olive), MPB (red) and post-MPB (blue). (a) Evolution of the Fe-L-edge fine structure; (inset) comparison of Fe-L edges for pre-MPB and MPB samples showing clear widening (spectra renormalized); (b) evolution of the O K-edge fine structure; pure BFO data (black) are added for comparison. Figure 4: NEXAFS data on Sm-substituted BFO samples with different compositions. Pre-MPB (olive), MPB (red) and post-MPB (blue). ( a ) Evolution of the Fe-L-edge fine structure; (inset) comparison of Fe-L edges for pre-MPB and MPB samples showing clear widening (spectra renormalized); ( b ) evolution of the O K-edge fine structure; pure BFO data (black) are added for comparison. Full size image The NEXAFS data above provide a coherent picture, together with the STEM results, of the distortion of the chemical bonding environment of the Bi–O–Bi and Fe–O–Fe due to the Sm substitution. To understand the observations, we note that structure of BFO is described by the a – a – a − tilt system, whereas the Pnma phase of SmFeO 3 is described by the a − a − a + (refs [19] , [20] ). It has been proposed that the bridging phase is associated with a new tilt system similar to that of NaNbO 3 stabilized through coupling of the octahedral rotations to antipolar Bi/Sm displacements. [20] The observations in Figs 2 and 3 suggest that the bridging phase is a complex interplay of polarization and strain. The octahedral tilt system likely acts as a means of coupling polar and structural degrees of freedom, with the modulated structure orientation driven by the preferred polarization direction in BFO. Changing lattice behaviour as the system moves towards and beyond the MPB induces substantial disturbances in local environment for oxygen, which is reflected in different EXAFS signatures. Despite the fact that MPB systems were first identified more than 50 years ago, many aspects of these materials remain unexplained. As stated before, the majority of the data was obtained for FE–FE MPBs; however, FE–AFE systems have very similar features, thus suggesting that similar mechanisms might be active. For FE–FE, scattering techniques often indicate the presence of low-symmetry monoclinic phases, giving rise to the concept of polarization rotation as the explanation for enhancement in dielectric/piezoelectric properties. However, polarization rotation is incompatible with the theory of phase transitions [12] . At the same time, the spatially resolved studies of these low-symmetry phases have revealed the presence of nanoscale textures formed by coexisting domains of different ferroic variants [32] , phases or compositional gradients with highly complex microstructures close to the MPB, which gets progressively simplified as one moves away in composition from the boundary [1] . In ferroelectrics and ferroelastics [12] , [33] , these textures have been described through the concept of adaptive phases, postulating that the energy of the domain wall vanishes as one approaches the MPB composition, resulting in the formation of nanometre scale structural domains. These domains are then described as the reason for the unique properties of MPB systems, as well as for the observed macroscopic monoclinic symmetries [34] . However, the formation of nanoscale twins, as well as adaptive phase formation in small volumes, remain unexplained, as well as multiple ordered phases observed in some MPB systems (for example, ref. 3 ) and the observed Raman signatures of the MPB systems [35] . Recently, it was pointed out that the addition of the flexoelectric interaction to the equation of state renormalizes all the polar, piezoelectric and dielectric properties of the system [36] , up to and including domain wall energy, which can then effectively become negative. While the notion of an interface with a negative energy is at the first glance paradoxical, similar concepts were previously used for description of incommensurate ferroic phases [37] , [38] , [39] , [40] , [41] , intercalation compounds [42] , [43] , crystallographic shear phases [44] and charge density waves. Essentially, an intrinsic wall instability predicts transition to the modulated phase where interfaces are uniformly distributed in space (that is, emergence of the long-range modulated phase as the thermodynamic ground state of the system), as opposed to formation of two-phase mixtures [45] , [46] , [47] . In particular, it was argued that the direct gradient coupling between the order parameters could lead to the oscillatory solutions and non-uniform pattern formation [47] . We note that the negative domain wall energy formalism is physically equivalent to considering the modulated phases as additional phases in the mix; however, here we choose to use the former approach as it deals explicitly with the modulation of structure and polarization. The present atomic level observation of the polarization and strain fields, that is, elementary order parameters, as reported here, provides insight into the structural phenomena at the MPB in the (Bi,Sm)FeO 3 system. We can thus examine our data for compatibilities with existing theories formulated for FE–FE MPBs. First of all, these observations show that the low-symmetry phase scenario suggested by Noheda et al . [11] is not applicable here, possibly because the concept of polarization rotation is not meaningful for FE–AFE boundaries. Second, we note that the observation of regular, pronounced modulations in the polarization and strain fields is inconsistent with the adaptive phase model of coexistent domains of different phases. Rather, the formation of the modulated structures as seen in Figs 2 and 3 is consistent with the behaviour of ferroics with negative wall energy, such as those in the incommensurate phases [37] , [38] , [39] , [40] , [41] . Here, we explore possible origins and implications of this behaviour. We note that the free energy for the AFE material can be represented as a sum of a classical 2-4-(6) Landau potential for polarization, P , and structural order parameter, A . The phase diagrams of the individual subsystems are well known (for example, for 2–4 potential a single solution with zero-order parameter above the transition temperature, and two symmetric non-zero solutions below). The coupled system with a biquadratic coupling [48] is remarkably more complex, but has been investigated in detail by Balashova and Tagantsev. [22] We further explore the potential origins of the observed domain wall instability, leading to the formation of spatially modulated periodic structures as the ground state of the system. We note that in our case the contributions of depolarization energy are not dominant, as from STEM data the polarization points predominantly in the direction along the domain walls. Thus, the scalar free energy containing the ferroelectric and structural 2–4 potentials, corresponding gradient terms, as well as quadratic coupling of the order parameters and the flexoelectric term (see Supplementary Discussion for full derivation) can be written as: Here A is the AFE order-parameter components, polarization P is the FE order parameter and u is the strain. We omit all tensorial notations for the sake of simplicity. The coefficients β ( T , y ) and α( T, y ) depend on temperature, T , and stoichiometry, y . Gradient coefficients g and v are taken to be positive for commensurate ferroics; w is positively defined. f is the flexoelectric coupling coefficient [49] , c is the component of the stiffness tensor and q is the electrostriction coefficient. The term ξ/2( P 2 A 2 ) is the quadratic coupling [48] between order-parameter fields (typical values of coupling constant ξ for Pb(Zr,Ti)O 3 (PZT) can be found in refs [50] , [51] ), while the term ξ∂ P /∂ xA 2 is the inhomogeneous flexoelectric coupling. Both terms are allowed by the general form symmetry (even in m 3 m ); note that terms such as P 2 ∂ A /∂ x are usually not allowed owing to the additional symmetry elements, associated with A (some translations in the case of anti-ferrodistortive transitions, etc.). Specifically, we note that the gradient term is renormalized by the flexoelectric effects as , [36] , [52] where s is the elastic compliance, and can potentially become negative. This suggests mechanisms for domain wall instability. While the associated parameters for BFO are unavailable, estimates for SrTiO 3 and PZT suggest that this effect can be very significant. For instance, using SrTiO 3 parameters, we could estimate the gradient term renormalization as and , where ×10 −11 V m 3 C −1 and ×10 −11 V m 3 C −1 . Note that g 44 =0.74 × 10 −11 V m 3 C −1 , g 11 is of the same order following Tagantsev et al . [52] Therefore could become negative for reasonable material parameters, in a sense making effective domain wall energy negative. The detailed analysis of the free energy (1) allows construction of the phase diagram as shown in Fig. 5a . The evolution of the free-energy surface proceeds from paraelectric ( P =0, A =0) to antiferroelectric ( P =0, A = A 0 ) and then to ferroelectric ( P =0, A =0) state. At the boundary of antiferroelectric and ferroelectric phases, the intrinsic modulated phase appears. Flexoelectric coupling controls the appearance of the modulated phase due to . The results of the numerical simulations of the evolution of the domain structure (plots of the two order parameters) for each phase in the diagram are given in Fig. 5b–e . In the paraelectric phase (I, Fig. 5b ) a=p =0; in the antiferroelectric structural phase (II, Fig. 5c ) a≠ 0, p =0. The mixed phase region (III, Fig. 5d ) exhibits modulated non-zero a and p , while the ferroelectric phase (IV, Fig. 5e ) has p≠ 0 and a= 0. Note that in the vicinity of the region III, the domain walls of the primary order parameter develop short-range modulation; the corresponding coherence length increases towards the centre, where a fully modulated phase is realized. 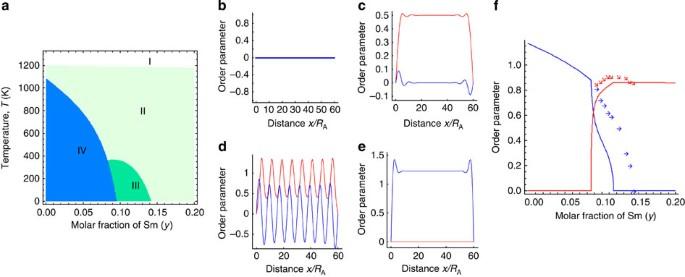Figure 5: Results of theoretical analysis for the model based on flexoelectric coupling. (a) Temperature versus Sm molar fraction phase diagram showing the areas of paraelectric (I), antiferroelectric (II), modulated (III) and ferroelectric (IV) phases. (b–e) Numerical simulations of the order parameter behaviour (a, red,p, blue) in the vicinity of the domain walls for (b) paraelectric phase (I) witha=p=0; (c) antiferroelectric structural phase (II) witha≠0, p=0; (d) mixed phase (III) with modulated non-zeroaandp; and (e) ferroelectric phase (IV) withp≠0,a=0. Other parameters, Δ=2,,,used in calculations are introduced in theSupplementary Discussion. (f) Room temperature section of the diagram across the MPB, with constant (solid lines) and oscillatory (arrows) components of the structural (a, red) and polarization (p, blue) order parameters plotted across the bridging phase region. Figure 5: Results of theoretical analysis for the model based on flexoelectric coupling. ( a ) Temperature versus Sm molar fraction phase diagram showing the areas of paraelectric (I), antiferroelectric (II), modulated (III) and ferroelectric (IV) phases. ( b–e ) Numerical simulations of the order parameter behaviour ( a , red, p , blue) in the vicinity of the domain walls for ( b ) paraelectric phase (I) with a=p =0; ( c ) antiferroelectric structural phase (II) with a≠ 0 , p =0; ( d ) mixed phase (III) with modulated non-zero a and p ; and ( e ) ferroelectric phase (IV) with p≠ 0, a= 0. Other parameters , Δ=2, , , used in calculations are introduced in the Supplementary Discussion . ( f ) Room temperature section of the diagram across the MPB, with constant (solid lines) and oscillatory (arrows) components of the structural ( a , red) and polarization ( p , blue) order parameters plotted across the bridging phase region. Full size image A detailed plot of the evolution of the constant (solid lines) and oscillatory (dots) components of the structural and polarization order parameter across the MPB along the RT cross-section is given in Fig. 5f . In full agreement with experiments, the amplitude of structural modulations remains almost constant across the bridging phase range, while the amplitude of polarization modulation is greatly reduced as the composition approaches the FE–AFE MPB. Thus, the approach based on flexoelectric coupling reproduces the general form of the phase diagram and predicts the modulated structure as a new ground state. Furthermore, even the evolution of the individual order parameters in the vicinity of the FE–AFE MPB is correctly reproduced. We note that application of the Ginsburg–Landau–Devonshire (GLD) formalism for the analysis of ferroic phenomena is necessarily limited, particularly for the cases when characteristic dimensions approach the atomic scale. Specifically, for small modulation periods the lattice pinning effects will have a strong role. Based on comparison with systems such as ordered defects in strongly non-stoichiometric compounds, crystallographic shear systems [42] and staged intercalation compounds [43] , the description in terms of suitable lattice level model may be more appropriate. In particular, we note that even the simplest Ising model with next nearest interactions (minimal model for material with two order parameters) can lead to a plethora of ordered phases. While a mean-field phase diagram predicts only the existence of ferroic and antiferroic phases, numerical simulations predict a variety of ordered phases. In this respect, we note that this model predicts the existence of the ¼ ordered phase indeed observed for the A-site-substituted BFO [3] , [21] , [53] , [54] , [55] . To summarize, the present work reveals spatially resolved order-parameter fields and their evolution at a FE–AFE MPB for the first time, and provides direct evidence for intrinsic material stability leading to the formation of spatially modulated phases. We argue that formation of modulated phases with well-defined periodicity controlled by the lock-on of lattice instability on the underlying lattice is the intrinsic feature of these systems, and this modulated state represents the true ground state of the system. This instability is further equivalent to the negative effective domain wall energy between parent FE and AFE phases and their different ferroic variants, and is induced by flexoelectric coupling between the polarization and strain gradients at the domain walls. This approach appears to describe this FE–AFE MPB system better than extending either of the currently accepted concepts of monoclinic and adaptive phases developed for description of FE–FE boundaries, and suggests that some MPB systems should be described similarly to chemically modulated systems such as intercalation compounds and crystallographic shear structures. At the same time, the universality of the shape of the phase diagram with the bridging/transitional phases not only for other morphotropic AFE–FE, but also FE–FE systems, suggests that similar mechanisms can in some cases be active as driven by competition between the structural and polarization order parameters. The reasoning could also apply to other ferroic systems with gradient coupling interactions such as flexomagnetism. Furthermore, given the similarity between nanoscale phase phenomena driven by competition between different ground states [56] , the present work has implications for other materials including manganites exhibiting colossal magnetoresistance [57] and other cases of phase separation. Thin film growth The samples with different Sm concentration in epitaxial thin film form were grown by pulsed laser ablation [19] . In both cases, the film thickness (in growth direction) is about 200 nm. The films have multiple domain boundaries and defects at the interface (see Supplementary Fig. S1 ); films grown in similar conditions were previously shown to have substrate-independent properties [19] , and are thus assumed to be completely relaxed. This was also confirmed by lattice parameter measurements [58] . Scanning transmission electron microscopy HAADF STEM images were acquired using FEI Titan S 80–300 operated at 300 kV and equipped with CEOS aberration corrector (probe semiangle 27 mrad, inner detector angle 80 mrad, probe size ~0.7 Å) ( Fig. 1c ) and Nion UltraSTEM 60–100 operated at 100 kV corrector (probe semiangle 30 mrad, inner detector angle 80 mrad, probe size ~0.9 Å) ( Fig. 1b ). The images were quantified by measuring atomic positions directly from images, based on a recent approach developed for TEM [59] , [60] and then extended for STEM [23] , [24] , [27] . EXAFS Soft X-ray absorption spectroscopy was carried out in National Synchrotron Radiation Research in Taiwan and was performed by the total electron yield where the incidence beam current and the sample drain current were simultaneously recorded to normalize the obtained spectrum with beam intensity. The polarization-dependent measurement at Fe L-edge and O K-edge were performed without changing the measurement geometry. How to cite this article: Borisevich, A.Y. et al . Atomic-scale evolution of modulated phases at the ferroelectric–antiferroelectric morphotropic phase boundary controlled by flexoelectric interaction. Nat. Commun. 3:775 doi: 10.1038/ncomms1778 (2012).